In situX-ray diffraction monitoring of a mechanochemical reaction reveals a unique topology metal-organic framework Chemical and physical transformations by milling are attracting enormous interest for their ability to access new materials and clean reactivity, and are central to a number of core industries, from mineral processing to pharmaceutical manufacturing. While continuous mechanical stress during milling is thought to create an environment supporting nonconventional reactivity and exotic intermediates, such speculations have remained without proof. Here we use in situ , real-time powder X-ray diffraction monitoring to discover and capture a metastable, novel-topology intermediate of a mechanochemical transformation. Monitoring the mechanochemical synthesis of an archetypal metal-organic framework ZIF-8 by in situ powder X-ray diffraction reveals unexpected amorphization, and on further milling recrystallization into a non-porous material via a metastable intermediate based on a previously unreported topology, herein named katsenite ( kat ). The discovery of this phase and topology provides direct evidence that milling transformations can involve short-lived, structurally unusual phases not yet accessed by conventional chemistry. Mechanochemical reactions by milling or grinding have emerged as excellent, rapid and cleaner alternatives to conventional chemical synthesis in a number of areas, from nanomaterials and alloys to pharmaceuticals and metal-organic frameworks [1] , [2] , [3] , [4] . However, despite significant and rapid advances in synthetic scope and methoodology [5] , [6] , [7] , the mechanistic understanding of mechanochemical reactions has remained elusive [8] , [9] , [10] , creating a major obstacle for the development and optimization of attractive proof-of-principle laboratory experiments into viable large scale processes [11] . It has been proposed that continuous mechanical stress and impact in a mechanochemical reaction environment can give rise to unusual reactivity or intermediate phases different than those normally accessible using conventional chemistry [12] . So far, there has been very little evidence [13] in support of or against such expectations due to a lack of methods that would permit direct, real-time insight into the rapidly agitated environment of an operating ball mill. Recently, however, we presented the first methodology for time-resolved in situ powder X-ray diffraction (PXRD) monitoring of mechanochemical reactions [14] as they take place [15] , [16] . In principle, this synchrotron radiation-based methodology now offers a unique opportunity to monitor mechanochemical reaction pathways and potentially observe unusual intermediate crystalline or amorphous phases whose existence might otherwise be only proposed or deduced by non-direct methods. The initial target of our study, the popular sodalite topology (SOD) framework ZIF-8 is known to form readily from ZnO and 2-methylimidazole ( HMeIm ) by liquid-assisted grinding (LAG), that is, milling using a small amount of a liquid additive that facilitates reactivity ( Fig. 1a,b ) [5] , [6] , [7] . 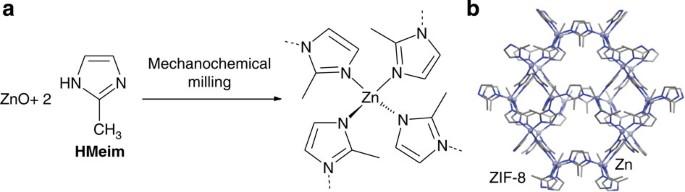Figure 1: Mechanosynthesis of ZIF-8. (a) Mechanochemical synthesis of ZIF-8; (b) Fragment of the crystal structure of ZIF-8. Figure 1: Mechanosynthesis of ZIF-8. ( a ) Mechanochemical synthesis of ZIF-8; ( b ) Fragment of the crystal structure of ZIF-8. Full size image Due to its high porosity and excellent resistance to pressure, temperature and steam, ZIF-8 has been extensively studied for applications in carbon sequestration and is also one the four metal-organic frameworks being manufactured commercially (Basolite Z1200) [17] , [18] , [19] , [20] , [21] , [22] , [23] , [24] , [25] . Crystallization of ZIF-8 from solution has been explored by several groups [26] , [27] , and a non-porous polymorph of ZIF-8 with a diamondoid ( dia ) topology was recently reported [28] , [29] . With the initial aim to simplify the mechanosynthesis of ZIF-8, which requires the presence of weakly acidic salts and an organic liquid (for example, N,N -dimethylformamide), we decided to explore LAG synthesis using only aqueous acetic acid. Here we report that in situ and real-time X-ray diffraction monitoring of mechanochemical ZIF-8 synthesis reveals an unexpected amorphization–crystallization process involving the intermediate formation of a previously not known metal-organic framework. The new framework is a metastable polymorph of ZIF-8, based on a hitherto unknown net topology, which we name katsenite ( kat ), demonstrating that monitoring of mechanochemical transformations in real time can reveal materials and structures that are difficult or even impossible to access by other means. Initial experiments The reaction mixture consisted of 0.8 mmol ZnO, 1.6 mmol HMeIm, giving a total of ≈200 mg of solid reactants and a designated volume of an aqueous solution of acetic acid with a concentration of either 2.50 or 1.25 mol dm −3 . The reaction mixture, along with two stainless-steel balls of 7-mm diameter (weight 1.3 g), was placed into an in-house designed 14 ml volume poly(methyl)methacrylate reaction jar and milled using a modified Retsch MM200 mill operating at 30 Hz ( Supplementary Fig. 1 ). The reaction was monitored in situ and in real time by diffraction of high-energy X-rays (87.4 keV, λ =0.14202 Å) at the European Synchrotron Radiation Facility (ESRF) Beamline ID15B [14] . For the initial experiment, conducted using 32 μl of 2.5 M aqueous acetic acid (~10 mol% acetic acid with respect to ZnO), the time-resolved diffractogram ( Fig. 2a ) revealed an almost immediate formation of ZIF-8, rapid disappearance of X-ray reflections of HMeIm and a much slower consumption of ZnO (see Methods, Supplementary Figs 2–7 ). Formation of ZIF-8 was recognized by its distinct PXRD pattern. Surprisingly, however, the intensity of X-ray reflections of ZIF-8 started to decrease after several minutes of milling. Within 40 min, the PXRD pattern exhibited only weak features of ZnO, indicating complete amorphization of the ZIF-8 formed initially. Such amorphization contrasts all previously reported mechanochemical LAG syntheses, where ZIF-8 was found to persist during milling [8] , [15] . Indeed, amorphization of ZIF-8 was previously reported only on dry milling of nano-sized crystals [30] , [31] , or on exposure to pressures >10 GPa (ref. 21 ). To elucidate the relative importance of the amount of acetic acid and the total volume of the liquid for the unexpected amorphization, the experiment was repeated, but using either half the amount of acetic acid in the same volume of liquid (32 μl of 1.25 M solution, Fig. 2b ) or using the same amount of acid, but in a larger volume of liquid (64 μl of 1.25 M solution, Fig. 2c ). 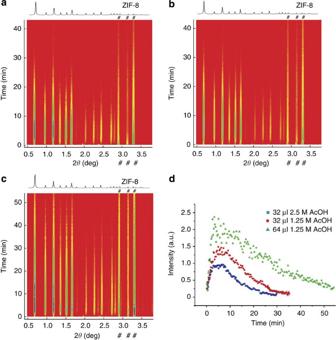Figure 2: Time-resolved diffractograms for the mechanochemical formation and amorphization of ZIF-8. Reactions were performed by milling ZnO andHMeImin the presence of aqueous acetic acid. The calculated PXRD pattern of ZIF-8 (CSD code VELVOY) is shown above each time-resolved diffractogram: (a) LAG with 32 μl of 2.5 M acetic acid (η=0.16 μl mg−1); (b) LAG with 32 μl of 1.25 M acetic acid (η=0.16 μl mg−1) and (c) LAG with 64 μl of 1.25 M acetic acid (η=0.32 μl mg−1). (d) The formation and amorphization of ZIF-8 illustrated by the change in intensity of the (011) reflection of ZIF-8, with error bars corresponding to s.d. In the time-resolved diffractograms, the reflections of ZnO starting material are highlighted by ‘#’. Selected examples and details of Rietveld analysis for experiments (a–c) are given in theSupplementary Figs 2–7andSupplementary Note 1. Figure 2: Time-resolved diffractograms for the mechanochemical formation and amorphization of ZIF-8. Reactions were performed by milling ZnO and HMeIm in the presence of aqueous acetic acid. The calculated PXRD pattern of ZIF-8 (CSD code VELVOY) is shown above each time-resolved diffractogram: ( a ) LAG with 32 μl of 2.5 M acetic acid ( η =0.16 μl mg − [1] ); ( b ) LAG with 32 μl of 1.25 M acetic acid ( η =0.16 μl mg −1 ) and ( c ) LAG with 64 μl of 1.25 M acetic acid ( η =0.32 μl mg −1 ). ( d ) The formation and amorphization of ZIF-8 illustrated by the change in intensity of the (011) reflection of ZIF-8, with error bars corresponding to s.d. In the time-resolved diffractograms, the reflections of ZnO starting material are highlighted by ‘#’. Selected examples and details of Rietveld analysis for experiments ( a – c ) are given in the Supplementary Figs 2–7 and Supplementary Note 1 . Full size image The results ( Fig. 2a–d ) reveal that the volume of liquid affects the amorphization of ZIF-8 more than the acid content: with 32 μl of aqueous acetic acid, complete amorphization of ZIF-8 was observed after ~30 min regardless of acetic acid concentration. With 64 μl of the 1.25 M solution, ZIF-8 was still clearly detectable after 55 min. Moreover, slow amorphization also took place with pure water as the grinding liquid, indicating that the weak acid facilitates, but is not mandatory for, the mechanically induced collapse of the ZIF-8 structure ( Supplementary Fig. 8 ). Properties of amorph -Zn(MeIm) 2 The amorphous material, designated amorph -Zn( MeIm ) 2 , could be dried in vacuum at room temperature or 40 °C and stored in a vial without recrystallization. Samples of amorph -Zn( MeIm ) 2 gave Brunauer-Emmett-Teller (BET) surface areas of 49–65 m 2 g −1 , indicating that the collapse of the initially formed open ZIF-8. The lack of porosity is consistent with the structure previously proposed for amorphous zinc bis(2-methylimidazole) on the basis of pair distribution function analysis [31] . Magic-angle spinning solid-state nuclear magnetic resonance measurements ( Fig. 3 ) on amorph -Zn( MeIm ) 2 revealed broad signals from three chemically distinct types of carbon atoms. The observed chemical shifts resemble those of ZIF-8, confirming the retention of a zinc imidazolate network, while the broadening of the NMR signals is consistent with the lack of long-range order. 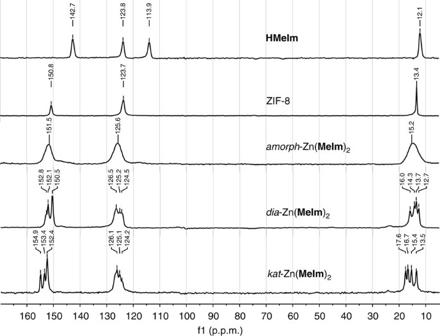Figure 3: CP-MAS13C SSNMR spectra. CP-MAS13C SSNMR spectra forHMeIm, ZIF-8,amorph-Zn(MeIm)2,dia-Zn(MeIm)2andkat-Zn(MeIm)2. The weak signal ~25 p.p.m. is assigned to the acetic acid additive in the reaction mixture. Figure 3: CP-MAS 13 C SSNMR spectra. CP-MAS 13 C SSNMR spectra for HMeIm , ZIF-8, amorph -Zn( MeIm ) 2 , dia -Zn( MeIm ) 2 and kat -Zn( MeIm ) 2 . The weak signal ~25 p.p.m. is assigned to the acetic acid additive in the reaction mixture. Full size image Discovery of a new phase Monitoring of mechanochemical reactions is affected by a changing and non-uniform distribution of the sample in the reaction vessel during milling, which results in scattering of the values of the measured diffraction intensity ( Fig. 2d ). To account for this effect, crystalline silicon (~20% by weight) was added into the reaction mixture as an internal scattering standard [32] . However, milling with silicon unexpectedly led to in situ recrystallization of the initial amorph -Zn( MeIm ) 2 after ≈30 min of milling, as shown by the appearance of reflections in the time-resolved diffractogram ( Fig. 4a,b ). The reflections did not correspond to either ZIF-8 or dia -Zn( MeIm ) 2 . Further milling led to the disappearance of these novel reflections and the appearance of reflections of the close-packed, non-porous dia -Zn( MeIm ) 2 (Cambridge Structural Database (CSD) OFERUN01, Supplementary Figs 9–13 ) [23] . 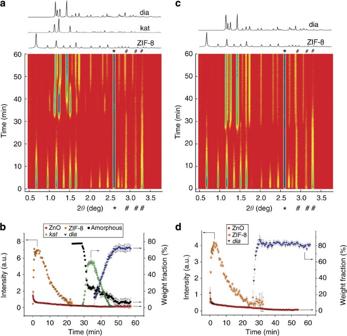Figure 4: Time-resolved diffractograms of mechanochemical amorphization and recrystallization. Mechanochemical LAG conversion of ZnO andHMeImin the presence of 2.5 M acetic acid with 20 wt% crystalline silicon as an internal scattering standard. The diffractogram (a) and the corresponding quantitative plot of the evolution of each phase (b) reveal the formation of the new (kat) phase at ~30 min milling. The diffractogram (c) and the corresponding quantitative plot for the evolution of each phase (d) demonstrate an experiment in which thekat-Zn(MeIm)2did not form anddia-Zn(MeIm)2crystallized directly from the amorphous phase. Final weight fraction of ~80% ofdia-Zn(MeIm)2for (d) indicates complete crystallization of the reaction mixture (remaining 20% being the silicon standard). Calculated PXRD patterns for crystalline phases are given on top of the time-resolved diffractograms. Due to the inability to establish the nature and arrangement of included guests in nascent ZIF-8, this phase was not included in Rietveld analysis. Instead, changes in the amount of ZIF-8 are represented with variations in the intensity of its (011) reflection, while changes in the amounts of other, non-porous phases are represented with variations of their weight fractions calculated by Rietveld analysis. Error bars correspond to s.d. obtained from the refinement procedure. To keep the liquid-to-solid ratio (η) after addition of silicon consistent with initial experiments, the volume of aqueous acid was 40 μl. Three characteristic ZnO reflections are marked with ‘#’, while the reflection of Si is marked with ‘*’. Examples of Rietveld analysis plots are given in theSupplementary Figs 9–13andSupplementary Note 1. Figure 4: Time-resolved diffractograms of mechanochemical amorphization and recrystallization. Mechanochemical LAG conversion of ZnO and HMeIm in the presence of 2.5 M acetic acid with 20 wt% crystalline silicon as an internal scattering standard. The diffractogram ( a ) and the corresponding quantitative plot of the evolution of each phase ( b ) reveal the formation of the new ( kat ) phase at ~30 min milling. The diffractogram ( c ) and the corresponding quantitative plot for the evolution of each phase ( d ) demonstrate an experiment in which the kat -Zn( MeIm ) 2 did not form and dia -Zn( MeIm ) 2 crystallized directly from the amorphous phase. Final weight fraction of ~80% of dia -Zn( MeIm ) 2 for ( d ) indicates complete crystallization of the reaction mixture (remaining 20% being the silicon standard). Calculated PXRD patterns for crystalline phases are given on top of the time-resolved diffractograms. Due to the inability to establish the nature and arrangement of included guests in nascent ZIF-8, this phase was not included in Rietveld analysis. Instead, changes in the amount of ZIF-8 are represented with variations in the intensity of its (011) reflection, while changes in the amounts of other, non-porous phases are represented with variations of their weight fractions calculated by Rietveld analysis. Error bars correspond to s.d. obtained from the refinement procedure. To keep the liquid-to-solid ratio ( η ) after addition of silicon consistent with initial experiments, the volume of aqueous acid was 40 μl. Three characteristic ZnO reflections are marked with ‘#’, while the reflection of Si is marked with ‘*’. Examples of Rietveld analysis plots are given in the Supplementary Figs 9–13 and Supplementary Note 1 . Full size image We subsequently established that the same unknown intermediate also appears in the absence of silicon, but only after longer milling (>50 min, Supplementary Figs 14–16 ). While it is tempting to conclude that crystallization of the new phase was facilitated by silicon acting as a heterogeneous nucleating agent, we found that the exact time of appearance of the new phase was difficult to reproduce, and that the crystallization of amorphous material sometimes directly gave dia -Zn( MeIm ) 2 ( Fig. 4c,d ). Such behaviour is characteristic of stochastic processes of nucleation from an amorphous matrix, and highlights the importance of in situ monitoring for the discovery of intermediate phases [33] . With the reaction course known, we were also able to reproduce the preparation of the new phase using conventional steel milling equipment in slightly over 50% of deliberate synthesis attempts, that is, the new kat phase was observed after milling in 9 out of 17 reactions (see Methods, Supplementary Fig. 17 ). Crystallization of amorph -Zn( MeIm ) 2 indicates a high degree of mobility imparted by wet milling, which contrasts its stability under storage and the earlier reports of stability of amorphized ZIF-8 under high pressures or dry milling [30] , [31] . As further evidence of the dynamic nature of the amorphous phase under milling conditions, we milled a dried sample of amorph -Zn( MeIm ) 2 with 100 μl of N,N -dimethylformamide, a solvent normally used for preparation of ZIF-8. Indeed, ZIF-8 was produced, indicating that amorph -Zn( MeIm ) 2 can be re-arranged back into the open SOD topology by wet milling in a suitable environment ( Supplementary Fig. 18 ). The katsenite topology The crystal structure of the new phase was solved from PXRD data ( Supplementary Fig. 19 , Supplementary Note 2 ) and revealed a new polymorph of Zn( MeIm ) 2 with a hitherto unknown framework topology which we named katsenite (three letter symbol: kat ). The new phase kat -Zn( MeIm ) 2 crystallizes in the tetragonal space group ( a =16.139(1) Å, b =16.321(1) Å) with four crystallographically independent Zn( II ) sites. Each Zn( II ) ion is in a tetrahedral environment defined by four 2-methylimidazolate ligands. Each ligand bridges two Zn( II ) ions to form a three-dimensional (3D) framework ( Fig. 5a ). Although this framework comprises only four-coordinated tetrahedral nodes, the underlying net is unique due to four non-equivalent 4-c nodes, each adopting a different coordination sequence and point symbol. Thus, we identified a quadrinodal network based on tetrahedral nodes with transitivity 4463 (see Methods, Supplementary Figs 20 and 21 , Supplementary Table 1 ). An augmented view of the kat -net, in which the nodes of the original net are replaced by their vertex figures, is shown in Fig. 5b . 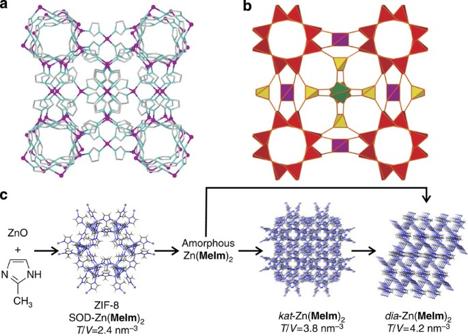Figure 5: Crystal structure and topology of katsenite and framework transformations. Structure ofkat-Zn(MeIm)2viewed along the crystallographicc-direction: (a) ball-and-stick representation and (b) thekatframework with different colouring for each type of vertex, represented by its vertex figure. (c) The sequence of solid-state transformations in the LAG reaction of ZnO andHMeIm: the transformations of ZIFs resemble the Ostwald's rule of stages33as they follow the order of increasingT/Vvalues, and hence the expected increase in the thermodynamic stability. Figure 5: Crystal structure and topology of katsenite and framework transformations. Structure of kat -Zn( MeIm ) 2 viewed along the crystallographic c -direction: ( a ) ball-and-stick representation and ( b ) the kat framework with different colouring for each type of vertex, represented by its vertex figure. ( c ) The sequence of solid-state transformations in the LAG reaction of ZnO and HMeIm : the transformations of ZIFs resemble the Ostwald's rule of stages [33] as they follow the order of increasing T / V values, and hence the expected increase in the thermodynamic stability. Full size image The new phase kat -Zn( MeIm ) 2 could be dried at room temperature in vacuum and stored for at least 3 months, which allowed a more extensive characterization and comparison to other zinc bis(2-methylimidazole) forms using thermogravimetric analysis and Fourier-transform infrared-attenuated total reflectance spectroscopy ( Supplementary Figs 22 and 23 ). Although stable at room temperature, kat -Zn( MeIm ) 2 readily rearranges into the dia phase by mild heating, for example, on attempted drying at 40 °C or on exposure to organic liquids(for example, on attempted washing with methanol). Consequently, samples of kat -Zn( MeIm ) 2 were investigated with minimum exposure to heat or washing. Examination of samples of amorph -, kat - and dia -Zn( MeIm ) 2 by scanning electron microscopy ( Supplementary Figs 24–26 ) did not reveal any significant differences in particle morphology. Attempts to use previously made kat -Zn( MeIm ) 2 to seed the recrystallization of amorph -Zn( MeIm ) 2 during milling were only partially successful, always yielding impure samples containing small amounts of ZIF-8. Tentatively, we rationalize the appearance of ZIF-8 impurity by epitaxial nucleation, due to the similarity of unit cell parameters between kat -Zn( MeIm ) 2 ( a =16.1 Å, c =16.3 Å) and ZIF-8 ( a =16.9 Å). The solid-state 13 C NMR spectrum of kat -Zn( MeIm ) 2 indicates four symmetrically non-equivalent MeIm − ligands, in agreement with the crystal structure obtained from X-ray powder diffraction data. Although the structure of dia -Zn( MeIm ) 2 also features four non-equivalent ligands, these two phases can be clearly distinguished by solid-state 13 C NMR chemical shifts of the ligand methyl groups ( Fig. 3 ). The structure of kat -Zn( MeIm ) 2 contains pores consisting of tight channels and pockets, which amount to 8% of the unit cell volume. Consistent with a low porosity structure, nitrogen gas sorption experiments revealed a low BET surface area of 37 m 2 g −1 for freshly prepared samples of kat -Zn( MeIm ) 2 dried in vacuum at room temperature. This is much less than that expected for a microporous material like ZIF-8 (without washing and activation, ZIF-8 prepared from ZnO in aqueous environment exhibits a BET surface area of ~1,300 m 2 g −1 ) [29] . Samples of dia -Zn( MeIm ) 2 prepared by mechanochemical collapse of ZIF-8 are non-porous, exhibiting an almost completely flat BET nitrogen sorption curve. The comparison of BET surface areas is consistent with the comparison of calculated densities for these materials: dia -Zn( MeIm ) 2 (1.578 g cm −3 ), kat -Zn( MeIm ) 2 (1.423 g cm −3 ) and ZIF-8 (0.922 g cm −3 ). The herein described crystalline→amorphous→crystalline transformation of ZIF-8 into its polymorphs kat -Zn( MeIm ) 2 or dia -Zn( MeIm ) 2 by milling in a water-containing environment is remarkable for several reasons. While amorphization on milling is a well-known phenomenon, spontaneous recrystallization of the mechanochemically obtained amorphous phase by continued milling has, to the best of our knowledge, not yet been described. Furthermore, the synthesis of crystalline ZIF-8 in aqueous solution has been described by several reports [34] , [35] , making the herein observed structural instability in the presence of water highly unexpected. Finally, previous studies [36] have consistently established that amorphous ZIF-8, which can be prepared either by neat milling of ZIF-8 or by exposing it to high pressures, does not rearrange into a crystalline material. Consequently, the observed transformation of amorph -Zn( MeIm ) 2 into different porous and non-porous crystalline frameworks is very much in contrast to established knowledge. It is, however, known that ZIFs are generally sensitive to acidic environments [37] and we believe that the observed transformations of ZIF-8 and of its amorphous form are the result of structural lability induced by a mildly acidic aqueous environment. The course of structural transformations observed taking place during milling is consistent with calculated order of stabilities with the dia -Zn( MeIm ) 2 being the most stable (see Supplementary Note 3 ). If dia -Zn( MeIm ) 2 is set as a reference point, kat -Zn( MeIm ) 2 is less stable by 0.16 kcal mol −1 (7 meV per atom) and ZIF-8 by 0.29 kcal mol −1 (12.7 meV per atom). The reaction course can also be more qualitatively rationalized by considering the number of tetrahedra ( T ) per volume ( V ) for each involved framework [38] . The T / V value of 3.8 nm −3 places kat -Zn( MeIm ) 2 between ZIF-8 ( T / V =2.4 nm −3 ) and dia -Zn( MeIm ) 2 ( T / V =4.2 nm −3 ). This reveals that the stepwise transformation of ZIF-8 into dia -Zn( MeIm ) 2 follows the Ostwald's rule of stages [33] and is driven by the formation of increasingly stable solid phases ( Fig. 5c ). Although the stepwise interconversion of ZIF-8 into kat -Zn( MeIm ) 2 and dia -Zn( MeIm ) 2 does not preserve any long-range topological features, a comparison of the secondary coordination sphere around crystallographically non-equivalent zinc nodes in kat -Zn( MeIm ) 2 reveals structural elements that are found in ZIF-8 and in dia -Zn( MeIm ) 2 , consistent with its role as an intermediate phase in the sequence SOD→ kat → dia . In conclusion, the presented results demonstrate the potential of in situ and real-time monitoring not only for understanding the processes taking place during milling, but also for the discovery of new phases and unexpected transformations in systems that are considered to be well-established. These results show that mechanical agitation under wet conditions provides means to access unconventional behaviour and structures different from those observed at static conditions or even under dry milling. In the context of understanding mechanochemical reactivity, the described results are an important advance as the first direct observation of an amorphization–recrystallization mechanism in mechanosynthesis and the first evidence of a metastable, structurally unusual intermediate in a mechanochemical process. The ability to use mechanochemical reaction monitoring to discover a new net topology in a system that has so far been subject to hundreds of studies is of outstanding importance in solid-state chemistry, and especially in the area of metal-organic frameworks [39] . Thus, our findings highlight the role of in situ and real-time PXRD monitoring as a complement to other experimental and computational studies of the structural landscape of metal-organic frameworks [40] , [41] . We note that the use of in situ monitoring to detect new phases appearing during milling may not be limited to metal-organic frameworks, but could very likely impact the understanding of structural transformations in related inorganic materials, such as zeolites and silicates, during mechanical processing or geological transformations [42] . Experimental set-up Real-time, in situ experiments were conducted at the ESRF beamline ID15B in a modified MM200 Retsch mill operating at 30 Hz [15] . The mill used was a Retsch MM200 ball mill with the sample holder custom modified to enable the access of the incident beam. Each reaction was conducted in a jar of 14 ml volume using two stainless-steel balls of 7-mm diameter (weight 1.33 g). Milling jars were fabricated so that the two complementary parts easily snapped together and did not leak liquid during the experiments [14] . The procedure of snapping the jar together and mounting it onto the mill was performed within 20 s or less, after which the milling was initiated by remote control and reaction course monitored in real time and in situ . The synthesis of kat -Zn( MeIm ) 2 , dia -Zn( MeIm ) 2 and amorph -Zn( MeIm ) 2 was reproduced outside the synchrotron facility using conventional equipment, that is, using a commercial Retsch MM400 mill operating at 30 Hz, with 200 mg of a mixture of ZnO and HMeIm in a stoichiometric ratio of 1:2 placed in a 10 ml stainless-steel jar along with a liquid additive and stainless-steel milling media. As milling media, we used either two 7 mm (each weighing 1.33 g) balls or a single 10-mm diameter ball (weight 4 g), with similar results. The formation of kat -Zn( MeIm ) 2 , dia -Zn( MeIm ) 2 and amorph -Zn( MeIm ) 2 was confirmed by PXRD analysis immediately after milling ( Supplementary Fig. 17 ). Reproducible synthesis of pure kat -Zn( MeIm ) 2 was challenging and the samples often contained a variable amount of dia -Zn( MeIm ) 2 . In contrast, the amorph -Zn( MeIm ) 2 was readily obtained by milling ZnO and HMeIm with either pure water or aqueous acetic acid ( c =2.5 M) for 30–50 min. Reproducible mechanosynthesis of dia -Zn( MeIm ) 2 was achieved by milling ZnO and HMeIm with1.25 M aqueous acetic acid for 90 min. Powder X-ray diffraction For in situ reaction monitoring, incident X-rays were selected using a bent Laue Si crystal, and the beam size on the sample was 300 × 300 μm 2 . Diffracted X-rays were detected with a flat panel Perkin-Elmer detector. Each diffractogram was typically obtained by summing 10 frames (or less), collected each with exposure time of 0.4 s, thus giving time resolution between successive diffractograms in seconds. The incident energy and detector distance (1,225.76 mm) were calibrated using a NIST CeO 2 standard sample and the Fit2D software package (ESRF Internal Report, ESRF98HA01T, FIT2D V9.129 Reference Manual V3.1, 1998). Raw data frames were integrated using Fit2D. For time-resolved 2D diffractograms the background for each pattern was subtracted using the Sonneveld–Visser [43] algorithm implemented in Powder3D [44] . Pawley [45] and Rietveld [46] refinements have been carried out on raw integrated diffraction patterns using Topas [47] . Laboratory PXRD experiments were conducted on a Bruker D2 Phaser equipped with a Cu K α X-ray source and a Ni filter. Reaction products with known crystal structures were identified by comparing the measured PXRD patterns to the ones simulated for known structures in the CSD (version 5.35, November 2013 update) or determined in this work. The structure of kat -Zn(MeIm) 2 The structure of kat -Zn(MeIm) 2 was solved by global optimization in direct space using the program Topas [47] , from PXRD data collected on a Bruker D8 Discovery X-ray diffractometer in the 2 θ range 5° to 65° using a Cu- K α ( λ =1.54 Å) source, equipped with a Våntec area detector and a nickel filter. The X-ray tube was operating at the power setting of 40 kV and 40 mA. Topological analysis was performed using the program TOPOS [48] . The structure is based on a 3D framework with an unprecedented topology and point symbol {4.7 3 .8 2 } 4 {4.7 4 .8} 2 {4 2 .7 4 }{7 4 .8 2 }. In the asymmetric unit, there are four crystallographically independent zinc ions (Zn(1), Zn(2), Zn(3) and Zn(4)), each in a tetrahedral environment defined by four nitrogen atoms of four different ligands. Although this new framework comprises only four-coordinated distorted tetrahedral nodes, the underlining network is unique due to the presence of four non-equivalent 4-c nodes, each adopting a different coordination sequence and point symbol ( Supplementary Table 1 , Supplementary Fig. 20 ). There are six kinds of non-equivalent essential rings: two 4-rings designated 4a and 4b ( Supplementary Fig. 21a ), two 7-rings and two 8-rings that are constructed by regarding the ligands as spacers between metal nodes. Vertices of the 4a -rings are alternating Zn(1) and Zn(3) nodes, while the 4b -rings are defined by Zn(2) nodes. The 4a -rings form infinite chains of corner-sharing rectangles by sharing Zn(3) nodes. The tetrahedral environment around each Zn(1) node in a 4a -ring is completed by two Zn(2) nodes. In that way, each 4a -ring in the kat structure is linked to four different 4b -rings. Finally, four 4b -rings connect to a Zn(4) node in a distorted tetrahedral arrangement. The above-mentioned arrangement of four-membered rings yields three different kinds of cages (tiles) with tiling [4 2 .8 2 ]+2[4.7 4 ]+2[7 4 .8 2 ] ( Supplementary Fig. 21b ). Before the final Rietveld refinement the structure model was optimized at 0 K in the space group P 1 using ab initio calculations ( Supplementary Note 2,3 ). Ab initio calculations Ab initio calculations of structural and electronic properties of all participating crystalline phases were performed using the VASP [49] code with the projector augmented wave method ( Supplementary Note 2,3 ) [50] . Consideration of van der Waals interactions was necessary to correctly evaluate relative stabilities of the investigated structures, namely, the density functional theory (DFT) calculations with self-consistently implemented van der Waals functional (vdW-DF) [51] , [52] , [53] give the order of stability in agreement with chemical behaviour and expectations based on differences in the density of tetrahedral centres. However, DFT calculations using general gradient approximation (GGA) type of the exchange correlation functional yield results that are clearly not consistent with the experiment, with relative energies of zinc(2-methylimidazolate) structures increasing in the order, that is, reverse from that expected: ZIF-8 [0]< kat -Zn( MeIm ) 2 (0.11 kcal mol −1 , 4.7 eV per atom)< dia -Zn( MeIm ) 2 (0.168 kcal mol −1 , 7.3 meV per atom). This demonstrates that in such situations [54] where total energies of investigated systems are close in value, the difference between results obtained with different functionals may not only be quantitative but also qualitative. Our results demonstrate that vdW-DF, as a nonlocal functional, is a better choice than the semi-local ones of the GGA type [55] . Accession codes : The X-ray crystallographic coordinates for the structure reported in this Article has been deposited at the Cambridge Crystallographic Data Centre (CCDC) under deposition number CCDC 989593. These data can be obtained free of charge from the CCDC via www.ccdc.cam.ac.uk/data_request/cif . How to cite this article: Katsenis A. D. et al . In situ X-ray diffraction monitoring of a mechanochemical reaction reveals a unique topology metal-organic framework. Nat. Commun. 6:6662 doi: 10.1038/ncomms7662 (2015).